Assessing the precision of morphogen gradients in neural tube development 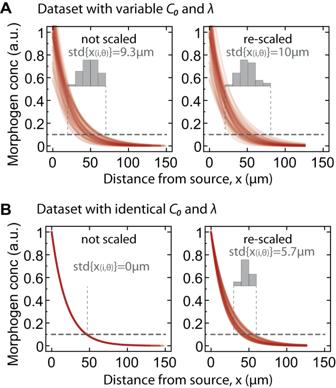Fig. 1: A numerical example of the rescaling error for exponential gradients with variableC0andλ. ALeft: Set of 50 randomly generated exponential morphogen profiles\(C\left(x\right)={C}_{0}{e}^{-x/\lambda }\). Meanλ= 20 µm andC0= 1.λandC0were varied by adding Gaussian noise with\(C{V}_{\lambda }\)= 0.2 and\(C{V}_{{C}_{0}}\)= 0.2. The domain length was randomly selected from uniform distribution between minL= 100 µm and maxL= 150 µm. 1 cell diameter (cd) = 4.9 µm (as in1). Dashed horizontal line indicates a concentration threshold\({C}_{\theta }\)= 0.1. At this threshold, the histogram of positions is shown, the mean position\({{{{{\rm{mean}}}}}}\{{x}_{i,\theta }\}\)is 48.4 µm from the source, and the positional error is\({{{{{\rm{std}}}}}}\{{x}_{i,\theta }\}\)= 9.3 µm = 1.90 cd. Right: The profiles are rescaled to the average length,\({{{{{\rm{mean}}}}}}\{{L}_{i}\}\)= 125.7 µm, by rescaling each\({\lambda }_{i}\)by a factor\({{{{{\rm{mean}}}}}}\left\{{L}_{i}\right\}/{L}_{i}\). In this set,\({{{{{\rm{mean}}}}}}\{{x}_{i,\theta }\}\)= 48.8 µm, and\({{{{{\rm{std}}}}}}\{{x}_{i,\theta }\}\)= 10.0 µm = 2.05 cd. This indicates that rescaling changed the positional error estimate\({{{{{\rm{std}}}}}}\{{x}_{i,\theta }\}\)by 0.15 cd.BIn Vetter and Iber, a scaling correction is estimated for exponential profiles without variability. A set of 50 such profiles is shown without and with rescaling (left and right, respectively). Assuming a uniform distribution of values at any given concentration threshold, the scaling error increases with distance to the source and reaches a maximum of 3 cd. Thus, the scaling error corresponds to\(3\xi\), where\(\xi\)denotes the relative position of the bin from the source. For the mean position at\({C}_{\theta }\)considered here (\({{{{{\rm{mean}}}}}}\left\{{x}_{i,\theta }\right\}\)= 46.7 µm),\(\xi\)= 46.7/125.7 = 0.37, hence the implied scaling correction is 1.11 cd ( = 5.4 μm). This is much higher than the rescaling error of 0.15 cd that we obtained for the dataset in A which incorporates realistic variability inC0andλ. Note that for an opposing gradient using the same coordinate system, the scaling correction should be 3(1-ξ). Yet, in Fig.2C, Eof Vetter and Iber2, the same correction of 3(1-ξ) is incorrectly applied to both the GBS-GFP and pSmad gradients. Had we used 3(1-ξ) as in2, the implied correction would be 1.8 cd and be even more overestimated compared to the actual rescaling error. 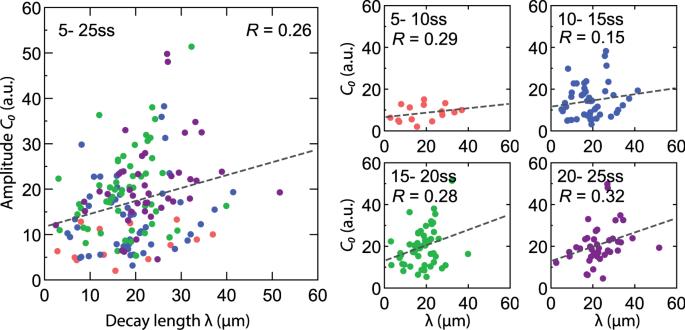Fig. 2: Correlation between the amplitudeC0and decay lengthλof measured Shh gradients. C0andλare obtained from exponential fits to the measured Shh ligand gradients from Cohen et al.11. Here, Shh profiles were assigned to developmental stages (designated ss for somite stage) based on their DV length as described in Zagorski et al. Dashed lines are linear fits to the data. For each stage, the Pearson correlation coefficient R is shown in the plot. For the pooled set of profiles between ss5 and ss25, the correlation coefficient is 0.26. Only stages up to 25ss are shown. Further information on research design is available in the Nature Portfolio Reporting Summary linked to this article.